Polycomb proteins control proliferation and transformation independently of cell cycle checkpoints by regulating DNA replication The ability of PRC1 and PRC2 to promote proliferation is a main feature that links polycomb (PcG) activity to cancer. PcGs silence the expression of the tumour suppressor locus Ink4a/Arf , whose products positively regulate pRb and p53 functions. Enhanced PcG activity is a frequent feature of human tumours, and PcG inhibition has been proposed as a strategy for cancer treatment. However, the recurrent inactivation of pRb/p53 responses in human cancers raises a question regarding the ability of PcG proteins to affect cellular proliferation independently from this checkpoint. Here we demonstrate that PRCs regulate cellular proliferation and transformation independently of the Ink4a/Arf-pRb-p53 pathway. We provide evidence that PRCs localize at replication forks, and that loss of their function directly affects the progression and symmetry of DNA replication forks. Thus, we have identified a novel activity by which PcGs can regulate cell proliferation independently of major cell cycle restriction checkpoints. Uncontrolled proliferation is one of the hallmarks of cancer that is required for tumour growth and spreading [1] . Normal cell cycle progression is tightly controlled by a variety of molecular checkpoints that supervise the biological processes that take place in the different phases of the cell cycle [2] . Notably, the cell cycle checkpoint that involves the Ink4a/Arf-p53-pRb axis has been described as the principle barrier to the initiation and maintenance of neoplastic transformation [3] , [4] , [5] , [6] . The crosstalk among the proteins active in these pathways and the epigenetic control of Ink4a/Arf expression have been widely investigated to characterize the role of proto-oncogenes that negatively affect this molecular checkpoint [7] , [8] . Among these, polycombs (PcGs) exert a fundamental role in controlling Ink4a/Arf transcriptional repression to promote cell cycle progression in physiological and pathological conditions [9] . PcGs pro-proliferative and oncogenic activities have been tightly linked with the transcriptional control of this locus, suggesting that PcG-dependent regulation of proliferation mainly depends on its ability to directly repress Ink4a/Arf expression [10] , [11] , [12] , [13] , [14] , [15] , [16] , [17] , [18] , [19] , [20] , [21] , [22] , [23] . Moreover, the PcG proteins Ring1b and Bmi1 can also directly regulate the p53 stability, further stressing their role in cellular proliferation and tumorigenesis by negatively acting on the pRb-p53 pathway [24] , [25] , [26] . In contrast, a few studies have also highlighted that the proto-oncogene Bmi1 can regulate proliferation independently of Ink4a/Arf expression [27] , [28] , [29] . Although the characterization of the overall role of PRC1 and PRC2 is incomplete, this finding suggests that additional mechanisms exist by which PcGs can regulate cellular proliferation. Several components of PRC1 and PRC2 are frequently overexpressed in human tumours and correlate with negative prognosis and poor survival [30] . Considering that the majority of tumours are also characterized by mutations in the Ink4a/Arf-p53-pRb axis [31] , we speculate that PcGs can affect cellular proliferation through additional mechanisms that acquire a particular significance during oncogenesis, thereby representing a potential therapeutic value [32] , [33] , [34] . Here we show that both PRC1 and PRC2 can regulate development, proliferation and transformation independently of the functionality of the Ink4a/Arf-p53-pRb pathway. We demonstrate that the genetic loss of PcG activity compromises the proliferation of both normal immortalized and fully transformed cells in the absence of major transcriptional changes. We provide evidence that PcG proteins are directly associated with replication forks, and that loss of PcG functions induce checkpoint-independent defects in the progression of DNA replication. PcG proteins are required for proliferation at low oxygen Mouse embryonic fibroblasts (MEFs), when placed in cell culture at atmospheric oxygen tension (normoxia, 21%), stop proliferating in a few passages and undergo oxidative-induced senescence. In contrast, when the same cells are grown at lower oxygen tension (hypoxia, 3% O 2 ), they grow indefinitely with no signs of senescence and maintain functional cell cycle restriction checkpoints [35] ( Fig. 1a,b ). However, in both conditions, cells accumulate similar levels of the two products of the Ink4a-Arf locus, namely, p19/Arf and p16 (ref. 35 ). This demonstrates that cells grown at low oxygen concentrations are insensitive to levels of p16 and p19/Arf that induce cell cycle arrest and senescence in normoxia conditions [35] . Based on this evidence, we hypothesized that loss of PcG repression would have a minor effect on the expression of the Ink4a-Arf locus at low oxygen tension (as locus expression is already activated in 3% O 2 cultures), and further, that loss of PcG activity would not have a major impact on the proliferation of cells grown at low oxygen concentrations. Thus, we analysed the role of PRC1 and PRC2 activity in the proliferation of mouse embryonic fibroblasts (MEFs) grown at low oxygen tension (3% O 2 ). Indeed, in contrast to normoxia (21% O 2 ), MEFs cultured in hypoxia (3% O 2 ) did not undergo stress-induced senescence, crisis and spontaneous immortalization but rather grew indefinitely ( Fig. 1a,b ). Consistent with previous reports [35] , our MEFs cultured at 3% O 2 accumulated p16 and p19/Arf levels to a similar extent as senescent cells grown at 21% O 2 without undergoing cell cycle arrest and senescence ( Fig. 1a,b ). At 3% O 2 , the expression of PRC2 and PRC1 components such as Ezh2, Suz12, Eed and Ring1b remained stable among the passages. In contrast, the PcGs levels in MEFs cultured at 21% O 2 reduced gradually with passaging while cellular senescence markers appeared ( Fig. 1a,b ), correlating the ability of cells to proliferate with an abundance of PcG proteins. In addition, strong differences in p53 activation were observed between normoxia and hypoxia conditions, consistent with previous reports [35] . 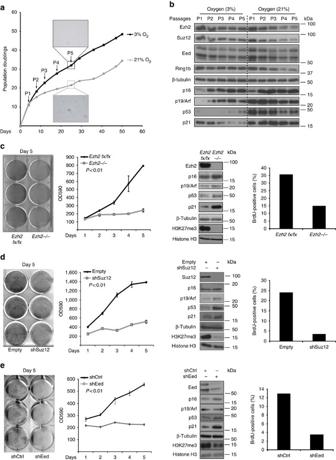Figure 1: PRC2 regulates MEF proliferation at 3% O2with high p16 and p19/Arf expression. (a) Cumulative population doublings of MEFs grown at 3% or 21% O2. Insets show a representative picture of the MEF stained for senescence-associated β-galactosidase activity (SA-β-gal) at passage 5. (b) Immunoblots using the indicated antibodies with protein extracts obtained from MEFs grown at 3 and 21% O2at the indicated passages. β-tubulin served as loading control. (c) Growth curves, immunoblots and BrdU FACS analysis ofEzh2 fx/fxandEzh2 −/−MEFs grown at 3% O2at the indicated time. Left panels show crystal violet staining of cells at day 5 of the growth curve. The graph represents the quantification of crystal violet absorbance atλ=590 nm at the indicated time points. Error bars indicate s.d.,n=3 for all graphs. Middle panel shows immunoblots using the indicated antibodies with protein extracts prepared fromEzh2 fx/fxandEzh2 −/−MEFs at day 5 of the growth curves. β-tubulin and total histone H3 served as loading controls. Bar plot in the right panel shows the percentage of BrdU incorporation as measured by FACS analysis betweenEzh2 fx/fxandEzh2 −/−MEFs. (d,e) As inc, using MEFs infected with Suz12- (d) or Eed- (e) specific shRNA-expressing lentiviral vectors. Empty or scrambled-expressing (ctrl) vectors were used as negative controls, respectively. Growth curves were performed at 3% O2. Figure 1: PRC2 regulates MEF proliferation at 3% O 2 with high p16 and p19/Arf expression. ( a ) Cumulative population doublings of MEFs grown at 3% or 21% O 2 . Insets show a representative picture of the MEF stained for senescence-associated β-galactosidase activity (SA-β-gal) at passage 5. ( b ) Immunoblots using the indicated antibodies with protein extracts obtained from MEFs grown at 3 and 21% O 2 at the indicated passages. β-tubulin served as loading control. ( c ) Growth curves, immunoblots and BrdU FACS analysis of Ezh2 fx/fx and Ezh2 −/− MEFs grown at 3% O 2 at the indicated time. Left panels show crystal violet staining of cells at day 5 of the growth curve. The graph represents the quantification of crystal violet absorbance at λ =590 nm at the indicated time points. Error bars indicate s.d., n =3 for all graphs. Middle panel shows immunoblots using the indicated antibodies with protein extracts prepared from Ezh2 fx/fx and Ezh2 −/− MEFs at day 5 of the growth curves. β-tubulin and total histone H3 served as loading controls. Bar plot in the right panel shows the percentage of BrdU incorporation as measured by FACS analysis between Ezh2 fx/fx and Ezh2 −/− MEFs. ( d , e ) As in c , using MEFs infected with Suz12- ( d ) or Eed- ( e ) specific shRNA-expressing lentiviral vectors. Empty or scrambled-expressing (ctrl) vectors were used as negative controls, respectively. Growth curves were performed at 3% O 2 . Full size image To test if PcG activity was required for MEF proliferation at low oxygen tension, we generated conditional knockout (cKO) MEFs ( Ezh2 fx/fx ) [36] under hypoxia conditions from mice that carried a 4-hydroxytamoxifen (OHT)–inducible oestrogen receptor fused to a CRE recombinase ( CRE-ER T2 ) that is constitutively expressed by the Rosa26 locus (R26) [37] . Contrary to our initial hypothesis, we observed that the proliferation of Ezh2 KO MEFs was strongly impaired at 3% O 2 after 1 week of OHT exposure, as shown by growth curves and BrdU incorporation assays ( Fig. 1c ), in the absence of any significant induction of cell death ( Supplementary Fig. 1A ). Similarly, knockdown of Suz12 and Eed (two essential PRC2 components [38] , [39] ) by stable expression of specific short hairpin RNAs also blocked MEF proliferation under hypoxia and reduced the BrdU incorporation levels ( Fig. 1d,e ). Importantly, loss of PRC2 activity only slightly increased p16, p19/ARF and p53 levels and upregulated p21 ( Fig. 1c–e ). p21 upregulation was not involved in the proliferation block induced by loss of PRC2 activity at 3% O 2 , as the shRNA-mediated knockdown of Suz12 expression in p21 –/– MEFs still impaired cellular growth ( Supplementary Fig. 1B ). Although these results suggest independency from Ink4a/Arf and p21 expression, they cannot exclude that pRb and p53 have a role in PRC2-dependent proliferation defects. Ink4a/Arf-p53-pRb-independent PRC2 proliferation control To test if PcG-dependent proliferation defects require p16 and p19/Arf expression, we crossed the R26Cre-ER T2 - Ezh2 fx/fx mice with an Ink4a/Arf –/– strain [5] and generated MEFs under hypoxia ( Supplementary Fig. 1C ). After 7 days of OHT exposure, loss of Ezh2 activity induced strong proliferation defects in the absence of a functional p16 and p19/Arf response ( Fig. 2a ). Similarly, tip-tail fibroblasts (TTF) derived from the same strain also had a compromised proliferation upon deletion of Ezh2 activity ( Supplementary Fig. 1D ). Consistent with this, the acute knockdown of Suz12 and Eed in Ink4a/Arf –/– MEFs further demonstrated that PRC2 affects proliferation independently of Ink4a/Arf expression at low ( Fig. 2b,c ) and atmospheric (data not shown) oxygen tension. 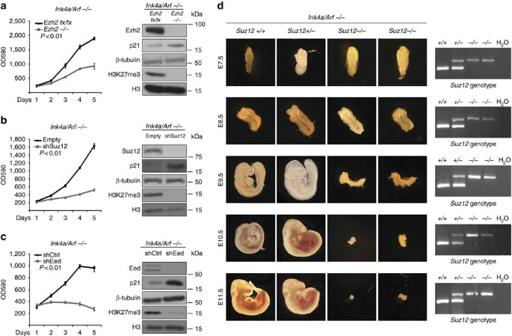Figure 2: PRC2 regulates proliferation and embryogenesis independently of Ink4a/Arf. (a–c) Growth curves measured with crystal violet (λ=590 nm, top panels) and western blot analysis of protein extracts using the indicated antibodies (bottom panels) fromEzh2 fx/fxandEzh2 −/− Ink4a/Arf −/−MEFs (left panels) orInk4a/Arf −/−MEFs infected with Suz12- (middle panels) or Eed- (right panels) specific shRNA-expressing lentiviral vectors grown at 3% O2. Empty and scrambled-expressing (ctrl) vectors were used as negative controls, respectively. Error bars indicate s.d.,n=3. (d) Pictures of embryos derived fromSuz12 +/−, Ink4a/Arf −/−mating at the indicated developmental stages. PCR genotypes of the single embryos at each developmental stage are presented in the right panels. Figure 2: PRC2 regulates proliferation and embryogenesis independently of Ink4a/Arf. ( a – c ) Growth curves measured with crystal violet ( λ =590 nm, top panels) and western blot analysis of protein extracts using the indicated antibodies (bottom panels) from Ezh2 fx/fx and Ezh2 −/− Ink4a/Arf −/− MEFs (left panels) or Ink4a/Arf −/− MEFs infected with Suz12- (middle panels) or Eed- (right panels) specific shRNA-expressing lentiviral vectors grown at 3% O 2 . Empty and scrambled-expressing (ctrl) vectors were used as negative controls, respectively. Error bars indicate s.d., n =3. ( d ) Pictures of embryos derived from Suz12 +/−, Ink4a/Arf −/− mating at the indicated developmental stages. PCR genotypes of the single embryos at each developmental stage are presented in the right panels. Full size image To gain in vivo insight for these observations, we took advantage of the Suz12 KO mouse model that we had previously generated [38] . Suz12 –/– embryos are blocked in embryonic development and die around 8.5 days post coitum (dpc) with strong proliferation defects [38] . We crossed Suz12 +/– mice into an Ink4a/Arf –/– background and tested whether loss of Ink4a/Arf expression could rescue its developmental and proliferative defects. Consistent with the results obtained with MEFs, the embryonic development of Suz12-Ink4a/Arf double KO embryos remained impaired, with a complete size block at 8.5 dpc ( Fig. 2d and Supplementary Fig. 1E ). Although we cannot discern the contribution between proliferation and differentiation defects, this result highlights in vivo the Ink4a/Arf-independent proprieties of PRC2 activity and suggests that defective proliferation could play a role in the PRC2-dependent developmental defects. To further investigate the role of pRb and p53 pathways in PcG-dependent proliferation control, we knocked down Suz12 expression in p53- ( p53–/– ) or pRb ( pRb–/– ) deficient MEFs. This experiment demonstrated that the loss of PRC2 activity induced proliferative defects even in the absence of either pRb or p53 functional responses ( Fig. 3a,b ; Supplementary Fig. 2A,B ). Moreover, to exclude that the two ‘arms’ of the pathway could generate compensatory effects, we simultaneously inactivated p53 and pRb functions by expressing the Large T oncoprotein encoded by the simian virus 40 early region (SV40ER) in Ezh2 cKO MEFs [3] ( Supplementary Fig. 2C ). Also in this case, OHT-mediated deletion of the Ezh2 locus induced proliferation defects ( Fig. 3c,d ). Differently from cells with proficient cell cycle checkpoints, loss of Ezh2 activity did not induce a cell cycle arrest but rather a constant reduction in the proliferation rate of the MEFs ( Supplementary Fig. 2D ). Overall, these data demonstrate that PRC2 can regulate cellular proliferation independently from the Ink4a/Arf-pRb-p53 axis. 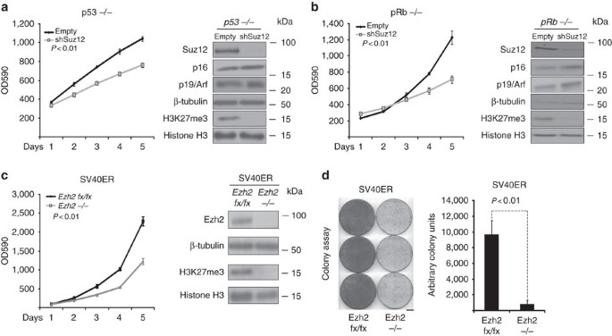Figure 3: PRC2 regulates proliferation in a p53- and pRb-independent manner. (a–c) Growth curves at 3% O2, measured with crystal violet (λ=590 nm, top panels) and immunoblots of protein extracts using the indicated antibodies (bottom panels) inp53−/−(a) andpRb−/−(b) MEFs infected with Suz12-specific shRNA-expressing lentiviral vectors, or SV40ER-immortalizedEzh2 fx/fxMEFs grown at 3% O2and treated with ethanol (Ezh2 fx/fx) or OHT (Ezh2 −/−). (c) An empty vector was used as a negative control for Suz12 knockdowns. β-tubulin and total histone H3 served as loading controls. Error bars indicate s.d.,n=3. (d) Colonigenic assay stained with crystal violet ofEzh2 fx/fxMEFs grown at 3% O2and treated with ethanol (Ezh2 fx/fx) or OHT (Ezh2 −/−). Colony quantification was determined using ImageJ. Error bars indicate s.d.,n=3.P-value was determined with pairedt-test. Scale bar, 2 cm. Figure 3: PRC2 regulates proliferation in a p53- and pRb-independent manner. ( a – c ) Growth curves at 3% O 2 , measured with crystal violet ( λ =590 nm, top panels) and immunoblots of protein extracts using the indicated antibodies (bottom panels) in p53−/− ( a ) and pRb−/− ( b ) MEFs infected with Suz12-specific shRNA-expressing lentiviral vectors, or SV40ER-immortalized Ezh2 fx/fx MEFs grown at 3% O 2 and treated with ethanol ( Ezh2 fx/fx ) or OHT ( Ezh2 −/− ). ( c ) An empty vector was used as a negative control for Suz12 knockdowns. β-tubulin and total histone H3 served as loading controls. Error bars indicate s.d., n =3. ( d ) Colonigenic assay stained with crystal violet of Ezh2 fx/fx MEFs grown at 3% O 2 and treated with ethanol ( Ezh2 fx/fx ) or OHT ( Ezh2 −/− ). Colony quantification was determined using ImageJ. Error bars indicate s.d., n =3. P -value was determined with paired t -test. Scale bar, 2 cm. Full size image PRC2 regulates transformation independently of p53-pRb PRC2 components are frequently found to be highly expressed in human tumours [30] , and this can be mirrored in cell culture using cellular immortalization and transformation protocols ( Supplementary Fig. 3A ). To assess whether the ability of PRC2 to regulate proliferation in a p53-pRb-independent manner could be a determinant for cellular transformation, we independently expressed the H-RASV12 and c-MYC oncogenes in R26Cre-ERT2, Ezh2 cKO MEFs that were previously immortalized by SV40ER expression ( Supplementary Fig. 2C ). First, we assayed the requirement of Ezh2 for the transformation of MEFs by expressing H-RASV12 or MYC in SV40ER-immortalized EZH2 –/– MEFs (condition defined as PRE). By performing colony and foci formation assays in cell culture or by inducing the in vivo formation of subcutaneous tumours in immunocompromised mice, we demonstrated that loss of Ezh2 activity prevented cellular transformation ( Fig. 4a–c , Supplementary Fig. 3B–E ). Consistent with this, when Ezh2 deletion was induced in MEFs that were already transformed by H-RASV12 or MYC expression (defined as POST), the neoplastic potential of these cells was strongly compromised both in cell culture and in in vivo transformation assays ( Fig. 4a,d,e , Supplementary Fig. 3D,F ). Together, these results demonstrate that Ezh2 is required for the transformation and maintenance of tumour growth even though the p53 and pRb pathways are inactivated. 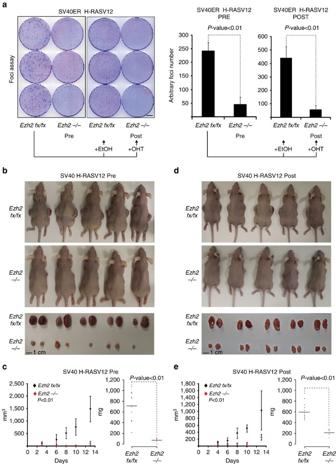Figure 4: PRC2 regulates cellular transformation in a p53- and pRb-independent manner. (a) Foci formation assay of SV40ER-immortalizedEzh2 fx/fxMEFs that stably expressed H-RASV12, treated with ethanol (Ezh2 fx/fx) or OHT (Ezh2 −/−). PRE indicates that SV40ER-immortalizedEzh2 fx/fxMEFs were exposed to OHT treatment before H-RASV12 expression. The POST condition indicates that H-RASV12 was expressed in SV40ER-immortalizedEzh2 fx/fxMEFs before OHT treatment. Foci were stained with Giemsa and quantified using ImageJ. Error bars indicate s.d.,n=3.P-value was determined with pairedt-test. All assays were performed at 21% O2. Scale bar, 2 cm. (b–e) Tumour formation of the cells described inaupon injection in both flanks of athymic nude mice. Pictures of nude mice and isolated tumour masses at 14 days post injection are shown inbandd; the average increase of tumour size at the indicated time (left) and the weights of the tumour masses (right) shown inbanddare given incande. Error bars indicate s.d.,n=10.P-value was determined using a Mann–Whitney test. Scale bars, 1 cm. Figure 4: PRC2 regulates cellular transformation in a p53- and pRb-independent manner. ( a ) Foci formation assay of SV40ER-immortalized Ezh2 fx/fx MEFs that stably expressed H-RASV12, treated with ethanol ( Ezh2 fx/fx ) or OHT ( Ezh2 −/− ). PRE indicates that SV40ER-immortalized Ezh2 fx/fx MEFs were exposed to OHT treatment before H-RASV12 expression. The POST condition indicates that H-RASV12 was expressed in SV40ER-immortalized Ezh2 fx/fx MEFs before OHT treatment. Foci were stained with Giemsa and quantified using ImageJ. Error bars indicate s.d., n =3. P -value was determined with paired t -test. All assays were performed at 21% O 2 . Scale bar, 2 cm. ( b – e ) Tumour formation of the cells described in a upon injection in both flanks of athymic nude mice. Pictures of nude mice and isolated tumour masses at 14 days post injection are shown in b and d ; the average increase of tumour size at the indicated time (left) and the weights of the tumour masses (right) shown in b and d are given in c and e . Error bars indicate s.d., n =10. P- value was determined using a Mann–Whitney test. Scale bars, 1 cm. Full size image Redundant role of PRC1 in proliferation and transformation The PRC1 complex regulates the same target genes as PRC2 and shares common biological functions with PRC2, and its recruitment to target gene promoters is, by large, dependent on H3K27me3 deposition [40] . Thus, we decided to investigate if the PRC1 complex also affects cellular proliferation in an Ink4a/Arf-pRb-p53-independent manner. We first measured the expression of Ring1b (the central catalytic subunit for all forms of PRC1) during MEF passages under hypoxic and normoxic conditions ( Fig. 1b ). We found that Ring1b expression was stable during passages under hypoxia but was downregulated during passages of MEFs grown under normoxia (for example, 21% O 2 ) as senescence occurred. Second, we generated R26Cre-ER T2 mice that carry a constitutively deleted allele for Ring1a ( Ring1a –/– , Supplementary Fig. 4A ) and a Cre-dependent conditional allele for Ring1b ( Ring1b fx/fx ) [41] . MEFs generated at 3% O 2 from these mice and exposed to OHT treatment for 1 week displayed a rapid cell cycle arrest ( Fig. 5a ). Compared with PRC2, loss of PRC1 activity induced a significant activation of p16 and p19/Arf expression that correlated with p53 stabilization and activation ( Fig. 5a ). This result suggests that PRC1 repression of Ink4a/Arf may be largely independent of PRC2 activity, and that the increased levels of p16 and p19/Arf could still induce a cell cycle arrest in Ring1a/b KO hypoxic cultures. Thus, we crossed these mice with an Ink4a/Arf –/– strain and tested if PRC1 activity was required for the proliferation of MEFs deficient in p16 and p19/Arf expression ( Supplementary Fig. 4B ). Consistent with our previous results, loss of PRC1 activity in Ink4a/Arf –/– MEFs impaired cellular proliferation under hypoxia conditions ( Fig. 5b ). To further exclude that pRb and p53 activation could still mediate a cell cycle arrest, we inhibited their activity by expressing SV40ER in Ring1a –/–, Ring1b fx/fx R26Cre-ER T2 MEFs ( Supplementary Fig. 2C ). As for Ezh2 KO MEFs, the inactivation of the Ring1b activity by OHT treatment inhibited cellular proliferation in the absence of a functional pRb and p53 pathway ( Fig. 5c ). 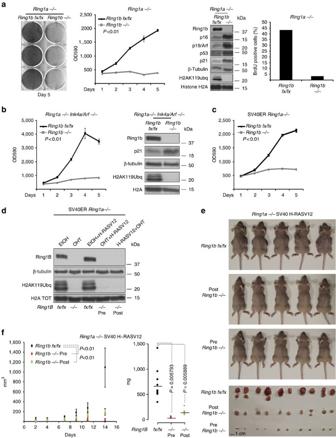Figure 5: PRC1 is required for proliferation and transformation independently of the Ink4a/Arf-p53-pRb axis. (a) Growth curves, immunoblots and BrdU FACS analysis ofRing1a −/−, Ring1b fx/fxandRing1a −/−andRing1b −/−MEFs grown at 3% O2for the indicated times. Left panels show the crystal violet staining of cells at day 5 of the growth curve. Quantification of crystal violet absorbance atλ=590 nm at the indicated time points is depicted in the graph. Middle panel shows immunoblots using the indicated antibodies of protein extracts derived fromRing1a −/− Ring1b fx/fxandRing1a −/−, Ring1b −/−MEFs at day 5. β-tubulin and total histone H2A served as loading controls. Right panel shows percentage of BrdU incorporation measured by FACS analysis betweenRing1a −/−,Ring1b fx/fxandRing1a −/−andRing1b −/−MEFs. In all growth curves, error bars indicate s.d.,n=3. (b) Growth curves and immunoblots as ina, usingInk4a/Arf −/−,Ring1a −/−,Ring1b fx/fxorRing1b −/−MEFs at 3% O2. β-tubulin and total histone H2A served as loading controls. (c) Growth curves as inawith SV40ER-immortalizedRing1a −/−orRing1b fx/fx MEFstreated with ethanol (Ring1b fx/fx) or OHT (Ring1b −/−) at 3% O2. (d) Immunoblots were performed with the indicated antibodies using protein extracts prepared from SV40ER-immortalizedRing1a −/−orRing1b fx/fxMEFs in which OHT treatment and H-RASV12 expression was combined with the order indicated in the figure. β-tubulin and total histone H2A served as loading controls. (e,f) Tumour formation of the cells described indby injection in both flanks of athymic nude mice. Pictures of mice and of the isolated tumour masses at 14 days post injection are shown ine. The average increase of tumour size at the indicated time (left) and the weights of the tumour masses shown ineare presented inf. Error bars indicate s.d.,n=10.P-value was determined using a Mann–Whitney test. Scale bar, 1 cm. Figure 5: PRC1 is required for proliferation and transformation independently of the Ink4a/Arf-p53-pRb axis. ( a ) Growth curves, immunoblots and BrdU FACS analysis of Ring1a −/−, Ring1b fx/fx and Ring1a −/− and Ring1b −/− MEFs grown at 3% O 2 for the indicated times. Left panels show the crystal violet staining of cells at day 5 of the growth curve. Quantification of crystal violet absorbance at λ =590 nm at the indicated time points is depicted in the graph. Middle panel shows immunoblots using the indicated antibodies of protein extracts derived from Ring1a −/− Ring1b fx/fx and Ring1a −/−, Ring1b −/− MEFs at day 5. β-tubulin and total histone H2A served as loading controls. Right panel shows percentage of BrdU incorporation measured by FACS analysis between Ring1a −/− , Ring1b fx/fx and Ring1a −/− and Ring1b −/− MEFs. In all growth curves, error bars indicate s.d., n =3. ( b ) Growth curves and immunoblots as in a , using Ink4a/Arf −/− , Ring1a −/− , Ring1b fx/fx or Ring1b −/− MEFs at 3% O 2 . β-tubulin and total histone H2A served as loading controls. ( c ) Growth curves as in a with SV40ER-immortalized Ring1a −/− or Ring1b fx/fx MEFs treated with ethanol ( Ring1b fx/fx ) or OHT ( Ring1b −/− ) at 3% O 2 . ( d ) Immunoblots were performed with the indicated antibodies using protein extracts prepared from SV40ER-immortalized Ring1a −/− or Ring1b fx/fx MEFs in which OHT treatment and H-RASV12 expression was combined with the order indicated in the figure. β-tubulin and total histone H2A served as loading controls. ( e , f ) Tumour formation of the cells described in d by injection in both flanks of athymic nude mice. Pictures of mice and of the isolated tumour masses at 14 days post injection are shown in e . The average increase of tumour size at the indicated time (left) and the weights of the tumour masses shown in e are presented in f . Error bars indicate s.d., n =10. P -value was determined using a Mann–Whitney test. Scale bar, 1 cm. Full size image To further test if PRC1 activity is required for the transformation of MEFs and tumour growth, we inactivated Ring1b before or after H-RASV12 ectopic expression (PRE and POST, respectively; Fig. 5d ). In both cases, colonies, foci formation and in vivo tumour growth was strongly inhibited by the loss of Ring1a and Ring1b functions, thus demonstrating that PRC1 is also essential for tumour growth independent of the pRb-p53 pathway ( Fig. 5e,f , Supplementary Fig. 4C–E ). These results were further supported by the rapid exhaustion of the self-renewing potential of normal and MYC-transformed hematopoietic stem cells upon inactivation of PRC1 activity ( Supplementary Fig. 4F ). Together, these results suggest the existence of alternative mechanisms of PcG-dependent regulation of proliferation that could be in common among different cell types. PcG proteins regulate S-phase entry and DNA replication Since PcGs repressive activity is not exclusively recruited at the Ink4a/Arf locus but potentially regulates the expression of more than 2,500 genes in MEFs ( Fig. 6a ), we hypothesized that additional proliferation-related genes could be under the direct transcriptional control of PcG proteins. To our surprise, expression analyses performed in Ink4a/Arf –/– Ezh2 –/– MEFs identified only 46 genes that were significantly upregulated upon loss of Ezh2 activity ( Fig. 6a ), despite the strong proliferation impairment displayed by these cells ( Fig. 2a ). In contrast, expression analyses performed in Ink4a/Arf +/+ Ezh2 –/– MEF identified 792 genes that were upregulated compared with Ezh2 fx/fx MEFs, of which only 31 were found commonly regulated between Ink4/Arf-proficient and KO MEFs ( Fig. 6a and Supplementary Table 1 ). Moreover, a low proportion of H3K27me3-enriched genes [42] (putative direct targets) was transcriptionally upregulated upon inactivation of Ezh2 activity in both wild-type and Ink4a/Arf –/– MEFs (~7% and ~0.4%, respectively). Finally, none of the proteins encoded by the genes upregulated in Ink4a/Arf –/– Ezh2 –/– MEFs retained known or putative functions that could suggest an indirect effect on cell proliferation. These data strongly suggest that the global transcriptional regulation induced by loss of Ezh2 in wild-type cells is likely a secondary event induced by checkpoint activation and arrest of the cell cycle ( Figs 2a and 6a ). Indeed, once depleted of Ezh2, Ink4a/Arf –/– MEFs only modestly regulated global gene expression and did not significantly activate PcG putative direct targets (9 out of 2,516), despite presenting strong proliferative defects ( Figs 2a and 6a ). Together, these data point towards a transcriptional-independent mechanism by which PcGs affect cellular proliferation. 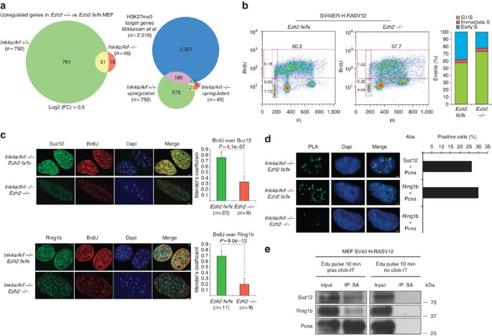Figure 6: PcGs regulate S-phase entry. (a) Venn diagrams representing the overlap of genes upregulated in eitherEzh2 fx/fxorInk4a/Arf −/− Ezh2 fx/fxMEF with OHT treatment (Ezh2 −/−) as compared with ethanol treatment (Ezh2 fx/fx), with a minimal fold difference of 1.5. The diagrams on the right represent the same overlap as previously characterized H3K27me3-enriched promoters in WT MEFs42. (b) FACS analyses of SV40ER-immortalizedEzh2 fx/fx MEFsthat stably expressed H-RASV12 7 days after ethanol (Ezh2 fx/fx) and OHT (Ezh2 −/−) treatment and fixed 30 min after release from a double-thymidine G1/S block in the presence of BrdU. The bar plots represent the relative percentage of cells with 2C DNA content present in the highlighted gates (BrdU negative, intermediate and BrdU positive). (c) Confocal immunofluorescence images ofInk4a/Arf −/−;Ezh2 fx/fxandInk4a/Arf −/− Ezh2 −/−MEFs 2 h after release from double-thymidine G1/S block following BrdU staining with the indicated antibodies. Bar plots indicate the average Mender’s colocalization coefficient among all images of the Z-stack for each cell. Error bars indicate s.d.nis indicated in the figure. Scale bars, 2 μm. (d) Proximity ligation assay co-incubating Suz12 and Pcna-specific antibodies inEzh2 fx/fx, Ink4a/Arf −/−(n=64) or by incubating Ring1b and Pcna-specific antibodies inEzh2 fx/fx, Ink4a/Arf −/−(n=50) or inEzh2 −/−,Ink4a/Arf −/−(n=46). (e) Accelerated native isolation of proteins on nascent DNA assay (aniPOND) performed in SV40, H-RASV12 transformed MEFs pulsed for 10 min with 10 μM of EdU. No Click-IT reaction served as negative control. Scale bars, 2 μm. Figure 6: PcGs regulate S-phase entry. ( a ) Venn diagrams representing the overlap of genes upregulated in either Ezh2 fx/fx or Ink4a/Arf −/− Ezh2 fx/fx MEF with OHT treatment ( Ezh2 −/− ) as compared with ethanol treatment ( Ezh2 fx/fx ), with a minimal fold difference of 1.5. The diagrams on the right represent the same overlap as previously characterized H3K27me3-enriched promoters in WT MEFs [42] . ( b ) FACS analyses of SV40ER-immortalized Ezh2 fx/fx MEFs that stably expressed H-RASV12 7 days after ethanol ( Ezh2 fx/fx ) and OHT ( Ezh2 −/− ) treatment and fixed 30 min after release from a double-thymidine G1/S block in the presence of BrdU. The bar plots represent the relative percentage of cells with 2C DNA content present in the highlighted gates (BrdU negative, intermediate and BrdU positive). ( c ) Confocal immunofluorescence images of Ink4a/Arf −/− ; Ezh2 fx/fx and Ink4a/Arf −/− Ezh2 −/− MEFs 2 h after release from double-thymidine G1/S block following BrdU staining with the indicated antibodies. Bar plots indicate the average Mender’s colocalization coefficient among all images of the Z-stack for each cell. Error bars indicate s.d. n is indicated in the figure. Scale bars, 2 μm. ( d ) Proximity ligation assay co-incubating Suz12 and Pcna-specific antibodies in Ezh2 fx/fx, Ink4a/Arf −/− ( n =64) or by incubating Ring1b and Pcna-specific antibodies in Ezh2 fx/fx, Ink4a/Arf −/− ( n =50) or in Ezh2 −/− , Ink4a/Arf −/− ( n =46). ( e ) Accelerated native isolation of proteins on nascent DNA assay (aniPOND) performed in SV40, H-RASV12 transformed MEFs pulsed for 10 min with 10 μM of EdU. No Click-IT reaction served as negative control. Scale bars, 2 μm. Full size image The loss of Suz12 expression from serum-starved quiescent human fibroblasts impairs the cell cycle re-entry, as measured by BrdU incorporation [38] . This result suggests that loss of PRC2 activity could affect the progression of G1 or S-phase. The finding that PcG proteins can remain associated with chromatin during DNA synthesis [43] , together with the localization of PRC2 subunits at sites of ongoing DNA replication [44] , potentially suggests a direct link between PcG activities and DNA replication. To test this, we synchronized Ezh2 fx/fx and Ezh2 –/– MEFs at the G1/S boundary with a double-thymidine block, allowed S-phase re-entry for 30 min in the presence of BrdU and measured DNA synthesis by flow cytometric analyses (FACS) with a BdrU-specific antibody. Due to the polyploidy of RASV12 or MYC-transformed MEFs [45] , [46] ( Fig. 6b and Supplementary Fig. 5A ), we restricted BrdU measurements to the 2C population to avoid cross-contaminations of G1/S boundaries. This analysis highlighted a reduced number of cells that synthesized DNA in Ezh2 –/– MEFs, suggesting direct defects of DNA replication in the absence of PRC2 activity ( Fig. 6b ). Consistent with this, Ezh2-proficient cells displayed a high degree of overlap between core PRC2 (Suz12) and PRC1 (Ring1b) subunits with sites of BrdU incorporation during S-phase ( Fig. 6c ). Loss of Ezh2 strongly reduced this colocalization, impairing Ring1b association with newly synthesized DNA ( Fig. 6c ). These results were further confirmed by proximity ligation assays using Suz12- or Ring1b-specific antibodies together with Pcna ( Fig. 6d ), an established marker of active DNA replication [47] . Consistent with the immunofluorescence results, we observed a distinct reduction of Ring1b association with Pcna in the absence of Ezh2 expression ( Fig. 6d ), strongly indicating a hierarchical recruitment at replication sites between PRC2 and PRC1 as described for several target genes [48] . Finally, to characterize the physical association of PcG proteins with sites of active DNA replication, we performed a native isolation of proteins on nascent DNA (aniPOND) [49] , demonstrating that components of PRC2 (Suz12) and PRC1 (Ring1b) directly associate with newly synthesized DNA in both wild-type ( Supplementary Fig. 5B ) and transformed cells (SV40-RASV12, Fig. 6e ). To test whether PcG deficiency could affect DNA replication, we performed DNA molecular combing experiments, which allow the quantitative study of individual DNA replication events [50] . Ezh2 fx/fx and Ezh2 –/– MEFs were pulse labelled with thymidine analogues, first with iododeoxyuridine (IdU) and then with chlorodeoxyuridine (CldU). DNA was purified and combed on glass slides, and IdU and CidU incorporation on newly synthesized DNA fibres was detected by fluorescent staining, together with anti-single-strand DNA antibodies. First, we measured the overall velocity of replication forks in the absence of Ezh2 activity and found that, while Ezh2-proficient MEFs displayed a unimodal fork speed distribution (centred around a mean fork velocity of 2.02 kb min −1 ), Ezh2 –/– cells displayed an overall slower velocity (mean velocity 1.79 kb min −1 ) and a bimodal distribution, highlighting the presence of a significantly slower DNA replication fork population ( Fig. 7a ). Similarly, reduced fork speed was also observed in PRC1-deficient MEFs ( Supplementary Fig. 5C ). Next, we determined the replication symmetry by measuring the length of newly synthesized DNA and comparing the progression of the left and right DNA replication forks departing in opposite directions from the same DNA replication origin. We observed three main patterns of DNA replication: ‘symmetric fork progression’ in which DNA replication fork progression is comparable between the left and right forks (with less than 30% difference, Fig. 7b top panel); ‘asymmetric fork progression’, in which the difference between the two DNA replication forks is more than 30% ( Fig. 7b middle panel); and ‘unidirectional fork progression’ in which only one DNA replication fork departs from one origin ( Fig. 7b , bottom panel). Following this classification, the analysis of replicating DNA from Ezh2 fx/fx and Ezh2 KO demonstrated that Ezh2 –/– MEFs accumulated a greater number of asymmetric and unidirectional DNA replication forks ( Fig. 7c ). 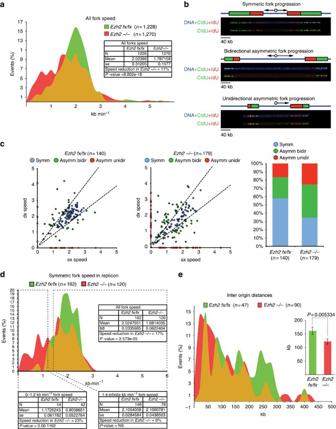Figure 7: PcGs supervise DNA replication. (a) Distribution of the replication speed for all forks between SV40ER-immortalizedEzh2 fx/fxMEFs that stably expressed H-RASV12 7 days after ethanol (Ezh2 fx/fx) or OHT (Ezh2 −/−) treatment.nis indicated in the figure.P-value was determined byλ2test. (b) Representative spinning disk confocal microscopy images of DNA combing performed in the cells presented inaand stained with the indicated antibodies. DNA fibres were visualized using ssDNA-specific antibodies. Scale bar, 40 kb. (c) Scatter plot of the fork distribution based on left/right fork speed ratio in the cells presented ina. Dotted lines indicate the 30% ratio tolerance applied to define symmetric fork progression. Box plots show the percentage distribution of fork symmetry betweenEzh2 fx/fxandEzh2 −/−cells described ina. (d) Distribution of replication speed for all symmetric forks forming a replicon betweenEzh2 fx/fxandEzh2 −/−cells described ina.nis indicated in the figure.P-value was determined byλ2test. (e) Distribution of inter-origin distances measured for all DNA fibres betweenEzh2 fx/fxandEzh2 −/−cells described ina. Bar plots show the average inter-origin distances ofEzh2 fx/fxandEzh2 −/−cells. Error bars indicate s.d.nis indicated in the figure.P-value was determined byλ2test. Figure 7: PcGs supervise DNA replication. ( a ) Distribution of the replication speed for all forks between SV40ER-immortalized Ezh2 fx/fx MEFs that stably expressed H-RASV12 7 days after ethanol ( Ezh2 fx/fx ) or OHT ( Ezh2 −/− ) treatment. n is indicated in the figure. P -value was determined by λ 2 test. ( b ) Representative spinning disk confocal microscopy images of DNA combing performed in the cells presented in a and stained with the indicated antibodies. DNA fibres were visualized using ssDNA-specific antibodies. Scale bar, 40 kb. ( c ) Scatter plot of the fork distribution based on left/right fork speed ratio in the cells presented in a . Dotted lines indicate the 30% ratio tolerance applied to define symmetric fork progression. Box plots show the percentage distribution of fork symmetry between Ezh2 fx/fx and Ezh2 −/− cells described in a . ( d ) Distribution of replication speed for all symmetric forks forming a replicon between Ezh2 fx/fx and Ezh2 −/− cells described in a . n is indicated in the figure. P -value was determined by λ 2 test. ( e ) Distribution of inter-origin distances measured for all DNA fibres between Ezh2 fx/fx and Ezh2 −/− cells described in a . Bar plots show the average inter-origin distances of Ezh2 fx/fx and Ezh2 −/− cells. Error bars indicate s.d. n is indicated in the figure. P -value was determined by λ 2 test. Full size image To test whether the reduction in fork speed was associated with asymmetric fork progression within individual replicons, we selected only the fork speed values derived from replicons, regardless of their levels of symmetry (all fork speeds in replicons, Supplementary Fig. 5D ). By analysing fork speed only in symmetric DNA replication operons (and thus excluding asymmetric ones), we observed a consistent reduction in fork speed in Ezh2 –/– MEFs as compared with wild-type MEFs (symmetric fork speed in replicons, Fig. 7d ). Overall, these results show that lack of Ezh2 increases the rate of DNA replication fork stalling, as demonstrated by increased levels of asymmetric and unidirectional forks. In addition, Ezh2 inactivation also reduces DNA replication fork speed, but, surprisingly, this is not restricted to only stalled (asymmetric) DNA replication forks. In yeasts, increased DNA replication fork stalling can trigger firing of dormant origins [51] . To test this possibility, we analysed the impact that loss of Ezh2 expression has on DNA replication origin firing. Accordingly to an increased impairment in DNA replication, Ezh2 KO cells showed an increased number of active replication origins, as inferred by the decreased inter-origin distances of Ezh2 –/– with respect to Ezh2 fx/fx cells ( Fig. 7e ). These differences were maintained also when the inter-origin distances was analysed on DNA fibres longer than three times the average fibres length [52] ( Supplementary Fig. 5E ). Furthermore, these results are not a consequence of increased DNA fibres fragmentation of Ezh2 KO samples, as both Ezh2 fx/fx and Ezh2 –/– DNA preparations displayed overlapping DNA length distribution ( Supplementary Fig. 5F ). Expression of oncogenes, such as RASV12, is known to infer a strong replicative stress to cells [53] . Consistent with a positive role in promoting DNA replication, Ezh2 requirement for cellular proliferation positively correlated with increased oncogenic pressure. In SV40-immortalized MEFs, loss of Ezh2 function resulted in a 1.88-fold proliferation reduction ( Fig. 8a,b ), but in H-RASV12-transformed MEFs (which grew 5.39-fold more than SV40-immortalized MEFs), the proliferation reduction was enhanced to 8.67-fold ( Fig. 8a,b ). These results underline the role of Ezh2 in sustaining the hyperproliferation that is frequently found in highly tumorigenic cells and highlight an important correlation between PcG activity and oncogene-induced replication stress. 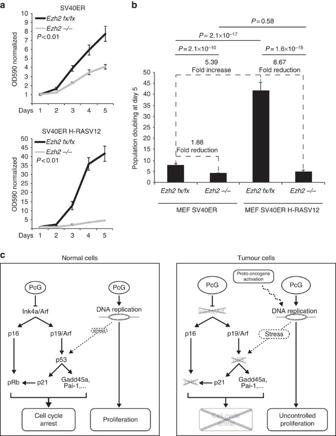Figure 8: Model of PcG regulation of cellular proliferation. (a) Normalized growth curves quantified by crystal violet staining of SV40 ER immortalized and SV40, H-RASV12-transformedEzh2 fx/fxMEFs treated with ethanol (Ezh2 fx/fx) or 4-OHT (Ezh2 −/−) for 7 days. Error bars indicate s.d.,n=3. (b) Bar plots indicating the number of population doublings after 5 days of growth curve calculated froma. Fold differences are indicated in the panel.P-values were determined by student'st-test. (c) The model highlights the role of PcGs in regulating DNA replication and cell cycle checkpoints in normal and neoplastic cells. Also, the frequent genetic deletions and oncogenic activities that occur in tumours cells are highlighted, to emphasize the requirement of PcG activities for the proliferation of cancer cells. Figure 8: Model of PcG regulation of cellular proliferation. ( a ) Normalized growth curves quantified by crystal violet staining of SV40 ER immortalized and SV40, H-RASV12-transformed Ezh2 fx/fx MEFs treated with ethanol ( Ezh2 fx/fx ) or 4-OHT ( Ezh2 −/− ) for 7 days. Error bars indicate s.d., n =3. ( b ) Bar plots indicating the number of population doublings after 5 days of growth curve calculated from a . Fold differences are indicated in the panel. P -values were determined by student's t -test. ( c ) The model highlights the role of PcGs in regulating DNA replication and cell cycle checkpoints in normal and neoplastic cells. Also, the frequent genetic deletions and oncogenic activities that occur in tumours cells are highlighted, to emphasize the requirement of PcG activities for the proliferation of cancer cells. Full size image Since altered DNA replication parameters, and in particular DNA replication stalling events, may activate the DNA damage response, we next monitored DNA damage response signalling at the single-cell level by studying 53BP1 foci formation in S-phase [54] . Ezh2-deficient MEFs present an increased number of 53BP1 foci with respect to wild-type cells ( Supplementary Fig. 6A ). Finally, consistent with a defective replication, PRC1-depleted cells displayed an increased level of damaged DNA, as demonstrated by a significant increase in tail moment detected in comet assays ( Supplementary Fig. 6B ). Overall, these data demonstrate that PcG activity localizes at sites of DNA synthesis and plays an important role in regulating the normal progression of DNA replication. In the present work, we provide genetic proof for the role of PRC2 and PRC1 in regulating normal and neoplastic cell proliferation independently of Ink4a/Arf-p53-pRb cell cycle regulation. This finding has a particular relevance in the context of tumour development, where loss of Ink4a/Arf , pRb and or p53 response is a hallmark for all type of human tumours [1] . Ezh2 enzymatic activity has become an appealing pharmacological target to stop tumour spreading [32] , [33] , [34] , and our data genetically support the effectiveness of PcG inhibition for cancer treatment. For example, it has recently been demonstrated that diffuse large B-cell lymphomas that carry hyperactivating mutations of Ezh2 (whereby diffuse large B-cell lymphomas frequently present defective p53 responses [55] , [56] ), can be efficiently treated with Ezh2-selective compounds [33] . Our findings suggest a scenario in which PcG proteins exert a parallel control over DNA replication and Ink4a/Arf transcription. Loss of PcG activities in normal cells will affect at the same time cellular proliferation, by favouring the efficient replication of the DNA, and cell cycle checkpoints, by regulating the transcription of Ink4a/Arf ( Fig. 8c ). While loss of Ink4a/Arf repression can activate cell cycle checkpoints, a defective DNA replication will trigger a parallel stress response to potentiate Ink4a/Arf-, pRb- and p53-dependent cell cycle arrest in a positive feedback loop ( Fig. 8c ). In the absence of functional checkpoints, cells will not undergo a cell cycle arrest, but their proliferation will still be dependent on PcG activity ( Fig. 8c ). An additional layer of complexity could come from PcG-dependent transcriptional regulation of additional targets. This could involve the de-repression of lineage-specific genes, which would thus be essential for the maintenance of cellular identity, or the activation of a common set of targets genes with anti-proliferative functions in all cell types. Although we cannot exclude these contributions, genome-wide transcription analysis performed in Ink4a/Arf –/– MEFs both before and after Ezh2 deletion did not show any relevant transcriptional effects despite their compromised proliferation ( Figs 2a and 6a ). Our data suggest that changes in gene expression detected in Ink4a/Arf-proficient cells (wild-type) upon inactivation of Ezh2 expression ( Fig. 6a ) are likely an indirect effect of cell cycle arrest rather than a loss of direct PcG repression of these genes. Indeed, the expression of the vast majority of H3K27me3-positive genes was unaltered in the absence of Ezh2 expression. Similarly, the majority of upregulated genes in Ezh2 –/– cells were not direct targets of PRC2 activity ( Fig. 6a ). These observations are consistent with recent studies performed in 293T cells (which express the SV40 T-antigen) that reported minor transcriptional changes upon loss of Suz12 expression [57] . It is likely that PcG repression of the Ink4a/Arf locus plays a crucial role in the proliferation of wild-type cells, thereby preventing checkpoint activation. However, our data clearly demonstrate that PcG proteins retain additional proprieties in regulating cell proliferation that do not involve genes’ transcriptional regulation. Tumour cells are exposed to continuous replication stresses imposed by the activity of oncogenic signals. Common examples are the constitutive activation of RAS signalling or the overexpression of the MYC proto-oncogene [53] , [58] . When replication stress is coupled to defective cell cycle checkpoints, it results in an escape from cellular senescence. At the same time, this prolonged replicative stress promotes the instability of cancer cell genomes [59] . This could suggest that the direct role in regulating DNA replication processes could render cancer cells more sensitive to PcG inhibition. The finding that PcG proteins colocalize and favour the progression of DNA replication suggests a direct implication of PcG activity with the replication of the DNA. PcGs could either play a role in origin firing, as depicted by the decreased inter-origin distance of Ezh2 –/– MEFs, or they could be involved in chromatin dynamics during the progression of the replication forks. Alternatively, PcGs could play a role in regulating the collision between RNA transcription and DNA replication, for example through their ability to bind to and disassemble the RNA polymerase II complex [60] . From our data, it is also clear that PcGs directly affect global fork speed independently of the degree of symmetry, indicating that they are required in general for fork progression and not exclusively in some stochastic events (for example, fork stalling). Nevertheless, it is possible that PcGs could be involved in promoting the progression of DNA replication in specific chromatin territories rather than exerting a global effect on replication. Together, our data provide evidence for a novel role of PcG proteins in regulating cellular proliferation that further explains the requirement of PcG activity for the growth of normal and cancer cells, paving the way for understanding novel mechanisms of PcG-dependent regulation of cellular proliferation. Ethics statement Experiments involving animals have been done in accordance with the Italian Laws (D.L.vo 116/92 and following additions), which enforces EU 86/609 Directive (Council Directive 86/609/EEC of 24 November 1986 on the approximation of laws, regulations and administrative provisions of the Member States regarding the protection of animals used for experimental and other scientific purposes). Mice have been housed accordingly to the guidelines set out in Commission Recommendation 2007/526/EC, 18 June 2007 on guidelines for the accommodation and care of animals used for experimental and other scientific purposes. MEF generation and growing conditions All MEFs were derived from 13.5 dpc embryos. Rosa26 CRE-ER T2 , Ezh2 knockout, Ink4a/Arf knockout, Suz12 knockout, p53 knockout, pRb knockout Ring1a knockout and Ring1b knockout genes used in this work have been described elsewhere [4] , [5] , [36] , [41] , [61] , [62] . In all experiments, low passages MEFs were grown in DMEM medium supplemented with 10% fetal bovine serum (Euroclone), non-essential amino acids (Gibco), sodium pyruvate (Gibco) and 1% penicillin/streptomycin (Gibco), in a CO 2 incubator (5% CO 2 ) with reduced oxygen tension (3% oxygen) if not otherwise specified. MEFs were passaged every 3–4 days. To induce CRE-ER T2 nuclear translocation, cells were treated with 500 nM of 4-hydroxytamoxifen (4-OHT, Sigma) dissolved in absolute ethanol (Panreac). For G1/S synchronization using a double-thymidine block, sub-confluent asynchronous MEFs were treated with 2 mM thymidine (Sigma) for 12 h, released with normal medium for 8 h and treated again with 2 mM thymidine for an additional 12 h. Beta-galactosidase staining MEFs (10 5 ) were grown in 3% oxygen or 21% oxygen (and 5% CO 2 ), plated at passage 5 (~20 days from derivation) on 0.1% gelatin-coated slide chambers and analysed for β-galactosidase positivity using the senescence β-galactosidase staining kit (Cell Signalling). Growth curves colony and foci formation assays Growth curves were performed by plating 5 × 10 4 cells per well in a 6-well plate, or 3 × 10 4 cells per well in a 12-well plate, in triplicate for each day of the growth curve. For daily measurements, cells were fixed in cold (4 °C) 4% formaldehyde buffered at pH 6.9 (Panreac) for 10 min at room temperature, washed twice with distilled water and air dried. At the end of each curve, single wells were stained with a 0.1% w/v solution of crystal violet (Sigma) for 30 min at room temperature. Plates were washed four times in water and dried overnight. Crystal violet was solubilized in 10% acetic acid (Carlo Erba), and absorbance measured at λ =590 nm. All growth curves were plated 1 week after OHT administration for the conditional knockout MEFs, and 2 days after antibiotic selection for the lentiviral-infected cells. Growth curves are representative of at least three independent experiments. Colony formation assays were performed with triplicate plating of 10 4 cells in a 10-cm dish. After 12–14 days, cells were fixed and stained with crystal violet as described above for growth curves. Foci formation was obtained by plating 4 × 10 6 SV40ER-immortalized MEFs with 2 × 10 5 SV40ER H–RASV12-transformed MEFs in a 10-cm dish. After 15–20 days, cells were fixed with 10% formaldehyde for 30 min at room temperature, stained with a 4% Giemsa (Sigma) solution in 1 × phsophate-buffered saline (PBS) for 2 h at room temperature, washed four times in water and air dried overnight. Foci formation assays are representative of at least two independent experiments. Colonies and foci counting were performed with ImageJ counting particle tools. Equal threshold settings and other parameters were applied to all images. Immunoblots For immunoblots, cells were lysed in 300 mM salt lysis buffer (20 mM Tris-HCl (pH 7.6), 300 mM NaCl, 5% glycerol, 0.2% Igepal). After lysis, the slurry was centrifuged at 13,000 r.p.m. for 15 min to pellet the material enriched in chromatin proteins that was not solubilized using 300 mM salt lysis buffer. Histones were purified from that pellet in 1% SDS, 9 M urea, 25 mM Tris-HCl (pH 6.8), 1 mM EDTA and 0.7 M mercaptoethanol. Following standard SDS–polyacrylamide gel electrophoresis (using different percentages according to the molecular weight of the proteins of interest), proteins were transferred to nitrocellulose membranes (Bio-Rad) and membranes were blocked in Tween 0.1% TBS (T-TBS), 5% milk powder overnight at 4 °C. Blocked membranes were then incubated in primary antibody diluted in blocking solution for 2 h at room temperature (for antibodies, see Supplementary Table 2 ), washed 3 × with T-TBS, and incubated for 1 h in secondary antibody diluted in blocking solution. Membranes were again washed 3 × with T-TBS, ECL (G&E Healthcare) was added to the membrane and the signal was detected on film (G&E Healthcare) [62] . All blots were carried out with protein lysates prepared 7–8 days after 4-OHT administration, or 2 days after antibiotic selection for the infected cells. Representative uncropped raw scans of blots generated with the most relevant antibodies used along the different figures are presented in Supplementary Figs 7–9 . BrdU FACS analysis Cells grown in the presence of 33 μM BrdU for the indicated time were fixed with 75% ethanol (Panreac), permeabilized with 2N HCl (Panreac) for 30 min at room temperature and pH equilibrated using 0.1 M BORAX (Sigma) for 2 min. Cells were incubated with a mouse anti-BrdU antibody (BD) in 1% BSA, 1 × PBS for 1 h at room temperature, washed and stained with a donkey anti-mouse FITC-conjugated antibody (Jackson). Stained cells were treated with RNase A (Sigma) followed by DNA staining with 2.5 μg μl –1 propidium iodide (Sigma) overnight at 4 °C. BrdU intensities were acquired by FACS Calibur and analysed using the FlowJo software. Antibody details are given in Supplementary Table 2 . Viral transductions Lentiviral transduction was carried out by infection with a VSV-G pseudotyped lentivirus. Viral particles were produced by calcium–phosphate transfection of 10 6 293T cells in a 10-cm dish using 10 μg of viral delivery vector, 3 μg of VSV-G and 6 μg of Δ8.2 packaging vectors per dish. After 36 h post transfection, the supernatant containing viral particles was collected, filtered at 0.45 μm and added to 5 × 10 5 MEFs that had been plated the day before on a 10-cm dish. Two rounds of infection (~8 h per day) were carried out for each plate in the presence of 5 μg ml –1 of polybrene (Sigma) followed by selection with the appropriate antibiotic selection. Retroviral transductions were carried out by transfecting 10 μg of the viral vector in 10 6 Phoenix-Eco cells plated on a 10-cm dish. Infections were carried out as for lentiviruses with the introduction of two additional round of infection (two per day) without polybrene. The vectors used for infections are listed in Supplementary Table 3 . Embryo development To obtain Suz12 –/– , Ink4a/Arf –/– double KO embryos, Suz12 +/– and Ink4a/Arf –/– were mated, and embryos analysed at the indicated time from the detection of vaginal plugs (referred as 0.5 dpc). The morphology of each embryo was recorded with a stereomicroscope and genotyped as previously described [61] . Nude mice tumour formation 10 6 cells were subcutaneously injected in each flank of 6-week-old female nude athymic mice ( nu/nu ) (Charles River laboratories) in 100 μl of 1 × PBS. Mass growth was measured every 2–3 days from the injection using an electronic caliper. Mice were killed after 14–15 days from injection and the tumour masses were isolated and weighed using an electronic scale. Immunofluorescence Indicated MEFs were seeded on 0.1% gelatinized glass coverslips and treated as indicated. To prepare nuclei on coverslips, cells were treated with cold pre-extraction buffer (10 mM Tris-HCl pH 7.6, 100 mM NaCl, 2 mM MgCl 2 , 0.3 M sucrose and 0.25% Igepal) for 10 min at 4 °C. Nuclei were fixed at –20 °C with 100% methanol (Panreac) for 10 min. Nuclei were further incubated with 20 mU μl –1 of DNaseI (NEB) for 30 min at 37 °C to unmask incorporated BrdU. Fixed nuclei were incubated with primary antibodies diluted in 0.1% Tween-TBS for 1 h at room temperature, washed and incubated with secondary antibodies conjugated with different fluorophores. Nuclei were counterstained with 4',6-diamidino-2-phenylindole and embedded in anti-fade glycerol (DABCO). Images were acquired using a Leica SP2 confocal microscopy. Mender’s colocalization coefficient was calculated on the entire images, Z-stacks, using the JACoP tool of the ImageJ software. Antibodies and reagents are listed in Supplementary Table 2 . Microarray expression analyses RNA from two independent OHT or ethanol treatments of Ezh2 fx/fx Ink4/Arf –/– MEF, and the RNA from one OHT or ethanol treatment in MEF Ezh2 fx/fx were hybridized independently to Mouse Gene 1.0 ST Affymetrix Arrays. Signals were RMA-normalized and analysed using Affy and limma bioconductor packages in R. Affy IDs were annotated using the mogene10sttranscriptcluster.db package. Probeset with a log2(FC) >0.5 expression difference and a P- value less than 0.05 were considered as differentially expressed. The microarray data have been deposited in the GEO database (GSE48520). DNA combing DNA combing was performed as previously described [50] , [64] . Briefly, cells were sequentially labelled for 20 min with 25 μM IdU followed by 20 min of 200 μM CldU incubation in the cell culture medium [64] . Labelled cells were embedded in agarose plugs, proteinase K-treated, DNA extracted and combed on silanized coverslips. DNA fibres were incubated with a mouse anti-ssDNA antibody (MAB3034, Chemicon) followed by anti-mouse IgG2a Alexa 546 coupled secondary antibody staining (Molecular Probes). Incorporation of halogenated nucleotides was detected with specific antibodies (IdU: mouse anti-BrdU, Becton Dickinson; CldU: rat anti-BrdU, Abcam) and visualized with appropriate secondary antibodies (goat anti-mouse IgG1-Alexa Fluor 647, Molecular Probes; goat anti-rat- Alexa Fluor 488, Molecular Probes). Images were acquired automatically with a spinning disk confocal microscope, and the individually labelled DNA molecules were manually measured with ImageJ. Antibodies used in the analyses are listed in Supplementary Table 2 . Comet assay The comet assay was performed on Ring1a –/– ; Ring1b fx/fx R26CRE-ER T2 MEF and Ring1a –/– ; Ring1b fx/fx R26CRE-ER T2 7 days after treatment with ethanol or 4-OHT, using a commercially available kit from Trevigen, 4250-050-K and following the neutral assay protocol. aniPOND Accelerated native isolation of proteins on nascent DNA (aniPOND) has been carried out as described by Leung KH et al. [49] Briefly, wild-type and SV40, H-RASV12-transformed MEF (around 3 × 10 7 cells for each experimental condition) were pulsed with 10 μM of EdU (Life technologies, A10044) for 20 or 10 min, respectively. Click-IT reaction was performed using biotin azide (Life Technologies, B10184) or dimethylsulphoxide as a negative control. Chromatin was sonicated following the procedure described by Leung KH et al. [49] Biotinylated Edu was captured overnight at 4 °C using streptavidin-coated magnetic beads (Life Technologies, 65602). Chromatin proteins bound to EdU were eluted and analysed by immunoblot. Proximity ligation assay Cells were prepared as described in the immunofluorescence section. The assay was developed following the manufacturer’s instructions (Duolink manual from Olink Biosciences). Briefly, cells were incubated with an anti-mouse PLUS (Sigma, DUO92001) and an anti-rabbit MINUS (Sigma, DUO92005) for 1 h at 37 °C, washed twice and then incubated with the ligase mix for 30 min at 37 °C (Sigma, DUO92014). After the ligase reaction, cells were washed twice and then incubated with the polymerase reaction containing a green intercalating dye for 100 min at 37 °C (Sigma, DUO92014). Finally, cells were washed twice and stained with 4',6-diamidino-2-phenylindole staining to visualize the nuclei (see immunofluorescence description). Pictures were taken using confocal microscopy (see immunofluorescence description). Cells were considered positive if at least three dots per cells were observed after merging all images of the Z-stack. Hematopoietic stem cells and methylcellulose assay Bone marrow cells collected from the femur and tibia of Ring1a –/– ; Ring1b fx/fx R26CRE-ER T2 mice were subjected to lineage negative (Lin–) enrichment using the hematopoietic progenitor enrichment kit (StemCell Technologies) to remove cells expressing differentiation antigens. Lin– cells were cultured in DMEM (Lonza) complemented with 10% fetal bovine serum for mouse myeloid colony-forming cells (scFBS StemCell Technologies), 100 ng ml –1 ) Stem Cell Factor (SCF) (Peprotech), 20 ng ml –1 recombinant IL3 (Peprotech), 20 ng ml –1 IL6 (Peprotech) and infected using a lentiviral-expressing vector EF1a-c-MYC. After two rounds of spin-infection using RetroNectin-coated plates and three days of 2 μg ml –1 puromycin selection, 5 × 10 3 Lin– cells were plated in each 35-mm dish and mixed with 1.2 ml of Metho cult GF M3434 (StemCell Technologies) in the presence of either 500 nM 4-OHT (Sigma) or ethanol (Panreac) as a control. After 7 days, colonies were counted and 5 × 10 3 cells derived from the colonies were re-plated two additional times in methylcellulose. Tip tail fibroblasts Mice Ink4a/Arf –/– ; Ezh2 fx/fx were killed, and 4–5 cm of the tail was cut and collected in cold 1 × PBS (Lonza). After sterilization (with ethanol), the tail was completely dried and incised with a razor for skin removal. The tail was diced in small pieces and then plated in six-well, 0.1% gelatin-coated plates in the same medium as described for MEFs. Statistical analyses Statistical analyses were carried out with R packages. P- values for growth curves and in vivo tumour growth were determined by computing the area under curve (AUC) using a kulife package applied for the Student's t -test between AUCs of two samples or groups. P- values for colonies and foci counts were generated using a paired t -test. P- values for tumour mass weights were generated using a Mann–Whitney test. P- values obtained for DNA combing analyses were determined with a λ 2 test. Accession codes : Microarray data for WT and Ink4a/Arf –/– MEFs with or without Ezh2 expression have been deposited in the NCBI Gene Expression Omnibus database under accession code GSE48520 . How to cite this article : Piunti, A. et al. Polycomb proteins control proliferation and transformation independently of cell cycle checkpoints by regulating DNA replication. Nat. Commun. 5:3649 doi: 10.1038/ncomms4649 (2014).